Highly stereoselective synthesis of cyclopentanes bearing four stereocentres by a rhodium carbene-initiated domino sequence Stereoselective synthesis of a cyclopentane nucleus by convergent annulation constitutes a significant challenge for synthetic chemists. Although a number of biologically relevant cyclopentane natural products are known, more often than not, the cyclopentane core is assembled in a stepwise manner because of the lack of efficient annulation strategies. Here we report the rhodium-catalysed reactions of vinyldiazoacetates with ( E )-1,3-disubstituted 2-butenols generate cyclopentanes, containing four new stereogenic centres with very high levels of stereoselectivity (99% ee, >97: 3 dr). The reaction proceeds by a carbene-initiated domino sequence consisting of five distinct steps: rhodium-bound oxonium ylide formation, [2,3]-sigmatropic rearrangement, oxy-Cope rearrangement, enol—keto tautomerization and finally an intramolecular carbonyl ene reaction. A systematic study is presented detailing how to control chirality transfer in each of the four stereo-defining steps of the cascade, consummating in the development of a highly stereoselective process. Construction of cyclopentanes constitutes an area of significant interest in the organic community [1] , [2] , [3] , as evidenced by numerous campaigns towards landmark natural products, including the prostaglandins [4] , [5] , [6] , [7] , [8] , [9] , [10] , [11] , [12] , [13] , [14] , [15] , [16] , jatrophanes [17] , [18] , [19] , [20] , [21] , [22] , [23] , [24] , [25] and pactamycin [26] , [27] . Synthetic cyclopentanes are a central motif common to prostaglandin antagonist antiglaucoma agents [28] , [29] , [30] , [31] , [32] . Indeed, the convergent, asymmetric synthesis of a cyclopentane nucleus bearing multiple chiral centres presents a distinct challenge for modern synthetic chemists. A general difficulty for a [3+2]-cycloaddition approach is developing a mild protocol to render a transient carbon dipole. One of the classic strategies for chiral cyclopentene synthesis involves stereoselective cyclopropanation of a 1,3-diene, followed by vinylcyclopropane rearrangement [33] , [34] , [35] , [36] . Contemporary efforts have involved the coupling of a suitably activated olefinic motif with an all carbon (1,3) dipole bound to a chiral metal centre via a formal [3+2]-cycloaddition [37] , [38] , [39] , [40] . A significant advancement has been the enantioselective cycloaddition of palladated trimethylenemethane with electron-deficient alkenes developed by Trost et al. [41] , [42] , [43] Alternatively, Fu et al. [44] , [45] and Zhang et al. [46] have disclosed enantioselective variants of the Lu cycloaddition [47] , [48] , [49] , [50] , [51] , [52] , [53] implementing chiral phosphine catalysts. Although a number of methods are available, the development of complementary strategies for the rapid construction of complex cyclopentanes is nonetheless desirable. In this article, we describe a convergent, stereoselective synthesis of cyclopentanes with four stereogenic centres from an annulation cascade involving vinyldiazoacetates and chiral allyl alcohols. Moreover, a detailed analysis to account for correlations between starting material architecture and reaction efficacy is described. First-generation synthesis In a 2011 report, we described our initial attempts to synthesize complex cyclopentanes 3 by means of a cascade sequence [54] . The strategy involved the coupling of racemic 3,3-dimethyl allyl alcohols ( 2 ) and donor/acceptor-substituted Rh(II) carbenes [55] , [56] derived from vinyldiazoacetates 1 in the presence of the dual-catalyst system, Rh 2 (DOSP) 4 and Sc(OTf) 3 , shown in Fig. 1a . Implementing 1 Mol % of chiral Rh catalyst enabled a high-yielding preparation of a range of cyclopentanes 3 , containing four stereogenic centres, as single diastereomers. Although we were pleased with the general efficacy with which a high degree of structural complexity was introduced from readily available building blocks, the reaction was characterized by a significant shortcoming: the enantioselectivity for the synthesis of 3 was variable (68–92% ee). In this paper we describe our diagnosis of the stereochemical limitations in our initial study, and the logical design of a stereo-controlled cyclopentane 5 synthesis, as illustrated in Fig. 1b . 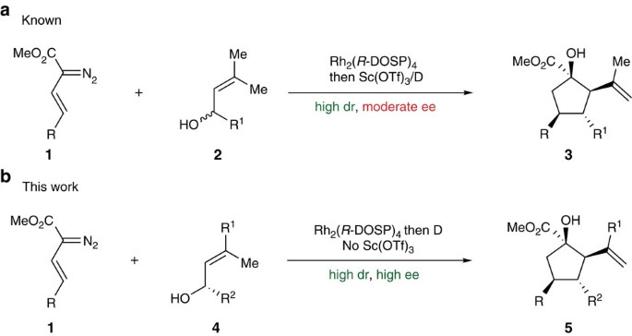Figure 1: Evolution of a Convergent Cyclopentane Synthesis. (a) One-pot synthesis of a cyclopentane (3) from a vinyldiazoacetate (1) and racemic allyl alcohol (2) in modest enantioselectivity via a rhodium-initiated cascade. (b) A second-generation cyclopentane (5) synthesis from analogous starting materials in high stereoselectivity. Figure 1: Evolution of a Convergent Cyclopentane Synthesis. ( a ) One-pot synthesis of a cyclopentane ( 3 ) from a vinyldiazoacetate ( 1 ) and racemic allyl alcohol ( 2 ) in modest enantioselectivity via a rhodium-initiated cascade. ( b ) A second-generation cyclopentane ( 5 ) synthesis from analogous starting materials in high stereoselectivity. Full size image Our previous synthesis of cyclopentane 3 involved four discrete, stereo-defining reactions, as illustrated for the specific example in Fig. 2 (ref. 52 ). The steps include: Rh-bound oxonium ylide formation ( 6 and 7 → I ), [2,3]-sigmatropic rearrangement ( I → 8 ) [55] oxy-Cope rearrangement ( 8 → II → 9 ) and intramolecular carbonyl ene reaction ( 9 → III → 10 ). Although the metal-bound ylide intermediate I is neither isolated nor observed in the tandem reaction, its intermediacy is well precedented in the literature [54] , [55] , [56] , [57] , [58] , [59] , [60] . From previous studies on the tandem ylide formation/[2,3]-sigmatropic rearrangement [61] as well as control studies [52] we have analysed the stereochemically relevant steps in the cascade sequence. We observed excellent enantiocontrol during the rhodium-catalysed process for generating the 3-hydroxy-1,5-hexadiene 8 (98% ee). Intermediate 8 then underwent a [3,3]-sigmatropic rearrangement through a chair-like transition state ( II ). Upon a subsequent enol—keto tautomerization, the product 9 , containing two new stereocentres, was furnished. The oxy-Cope rearrangement afforded a single diastereomer of ketoester 9 , an observation consistent with chair-like transition states being solely operative [52] , [61] , [62] , [63] , [64] . Isolation and chiral HPLC analysis of 9 , however, indicated partial racemization during the course of this step of the cascade sequence. The terminating sequence of the cascade—intramolecular carbonyl ene reaction via III —proceeded smoothly to furnish cyclopentane 10 as a single diastereomer. No further degradation in enantiopurity was observed during the ene reaction. These studies identify the origins of the moderate overall enantioinduction: modest chirality transfer during the oxy-Cope rearrangement. 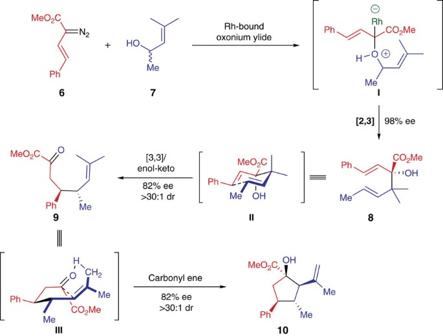Figure 2: Mechanism of cyclopentane synthesis. Mechanism of the one-pot domino sequence for the synthesis of a cyclopentane (10) from a diazoacetate (6) and a racemic allyl alcohol (7). Figure 2: Mechanism of cyclopentane synthesis. Mechanism of the one-pot domino sequence for the synthesis of a cyclopentane ( 10 ) from a diazoacetate ( 6 ) and a racemic allyl alcohol ( 7 ). Full size image Stereochemical limitations A rationale for the erosion in enantiopurity observed during the course of the oxy-Cope rearrangement is provided schematically in Fig. 3 . On the basis of cyclohexane A values, the equatorial versus axial positioning of carbomethoxy ( Fig. 3a ) and hydroxy ( Fig. 3b ) substituents would be favoured by 1.25 and 0.55 kcal mol −1 , respectively [65] . Equilibration between two possible chair-like intermediates for the [3,3]-sigmatropic rearrangement, shown in Fig. 3c , is more complicated. Both geminal disubstitution [66] and pseudoanomeric stabilization of the allyl hydroxy group [67] influence the equilibrium between IV and IV′ . On the basis of the A -values of the individual substituents and the psuedoanomeric stabilization-afforded IV , we can rationalize the modest preference for that pathway. Nevertheless, rearrangement via the energetically less favourable intermediate IV′ would also be feasible. Upon undergoing the Cope rearrangement, two of the stereogenic centres found in the cyclopentane ( 10 ), C(3) and C(4), have been installed. As can be seen from comparison of 9´ and ent -9´ , the competing chair-like transition states give rise to enantiomeric intermediates. Thus, enantiomers of the cyclopentane, 10 and ent -10 , arise from the competition between IV and IV′ . The 82% ee observed for the cyclopentane 10 synthesis is because of approximately a ten-to-one preference for IV over IV′ . 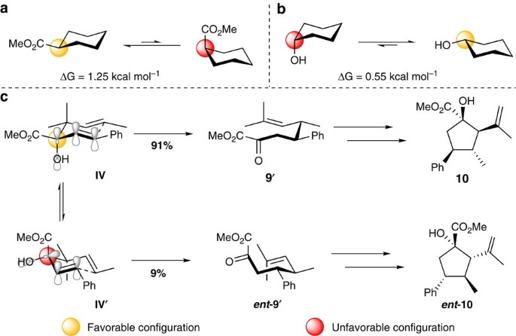Figure 3: Stereoelectronic considerations for an oxy-Cope rearrangement. CyclohexaneAvalues for carbomethoxy- (a) and hydroxy (b) -substituted cyclohexanes. (c) Manifestation of stereoelectronic effects in the competition between two chair-like transition states (IVandIV′). Figure 3: Stereoelectronic considerations for an oxy-Cope rearrangement. Cyclohexane A values for carbomethoxy- ( a ) and hydroxy ( b ) -substituted cyclohexanes. ( c ) Manifestation of stereoelectronic effects in the competition between two chair-like transition states ( IV and IV′ ). Full size image Rationale for second-generation synthesis Having analysed the reaction responsible for partial racemization in the cascade sequence, we honed our efforts towards a general solution to the problematic step. On the basis of the hypothesis that competing chair-like transition states during the oxy-Cope rearrangement were the source of poor chirality transfer, we designed new systems that would suppress this equilibration and strongly favour one chair-like transition state over the other. In a recent article, we described the tandem ylide formation/[2,3]-sigmatropic rearrangement of readily available chiral allyl alcohols with donor/acceptor-substituted rhodium carbenes 75 . For alcohols with variable substitution at C(3) ( Fig. 4a , 11 , R 1 ≠ R 2 ), rearrangement products bearing vicinal stereocentres ( 12 ) were generated with very high enantiocontrol (>99% ee) and moderately high diastereocontrol (12−>20: 1). Specifically, the rhodium catalyst dictated the configuration of the hydroxyester stereocentre (green sphere), while the allyl alcohol controlled the configuration of the second chiral centre (blue sphere). Thus, we demonstrated that the proper combination of each enantiomer of Rh 2 (DOSP) 4 and allyl alcohol enabled the synthesis of all four diastereomers of 12 . We envisioned that the [2,3]-sigmatropic rearrangement to generate a product with adjacent stereocentres could provide the necessary solution to chirality transfer during the problematic oxy-Cope rearrangement, as shown in Fig. 3b . Specifically, the proper configuration of a 3-hydroxy-1,5-hexadiene ( 12 ) would enable a single chair-like intermediate, wherein both chiral centres would orient cooperatively ( 12′ ), with the substituents having larger A -values positioned equatorially ( R 1 > R 2 ). Herein, we report the synthesis-based exploration of that hypothesis and the development of a highly stereoselective cyclopentane synthesis. 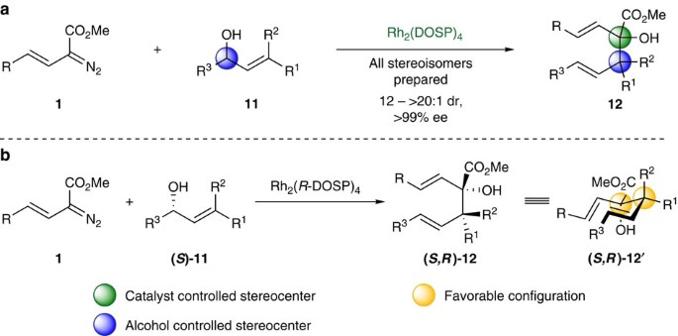Figure 4: Rationale for improved chirality transfer during an oxy-Cope rearrangement. (a) The tandem-ylide formation/[2,3]-sigmatropic rearrangement between a diazoacetate (1) and allyl alcohol (S)-11 (2) to generate a 3-hydroxy-1,5-hexadiene (12) bearing vicinal stereocentres and (b) application toward stabilization of a chair-like transition state. Figure 4: Rationale for improved chirality transfer during an oxy-Cope rearrangement. ( a ) The tandem-ylide formation/[2,3]-sigmatropic rearrangement between a diazoacetate ( 1 ) and allyl alcohol (S)-11 ( 2 ) to generate a 3-hydroxy-1,5-hexadiene ( 12 ) bearing vicinal stereocentres and ( b ) application toward stabilization of a chair-like transition state. Full size image Our investigations into an improved cyclopentane synthesis began with a series of control reactions. First, the diastereo- and enantiomerically pure 3-hydroxy-1,5-hexadiene 13 (ref. 75) was heated in a sealed tube for 12 h. Direct purification using flash chromatography afforded a small amount of the ketoester 14 as a single stereoisomer ( Fig. 5a ). The modest isolated yield of 14 is because the crude reaction mixture contains a mixture of starting material ( 13 ), ketoester ( 14 ) and cyclopentane ( 15 ). Prolonged heating of 13 furnished the desired cyclopentane 15 in excellent yield and with no loss in the level of enantioselectivity, as shown in Fig. 5b . The product 15 was, however, formed as an 88: 12 mixture of diastereomers. Having established that the keto ester 14 is formed as a single diastereomer, it appears that the carbonyl ene reaction to form 15 is no longer highly diastereoselective with these substrates. Comparison with literature precedent [22] and our own analyses of the nuclear Overhauser effects ( Supplementary Figs 1 and 2 ) in 15 are indicative of inversion in the configuration at the C(1)- and C(2) stereocentres in the minor product. 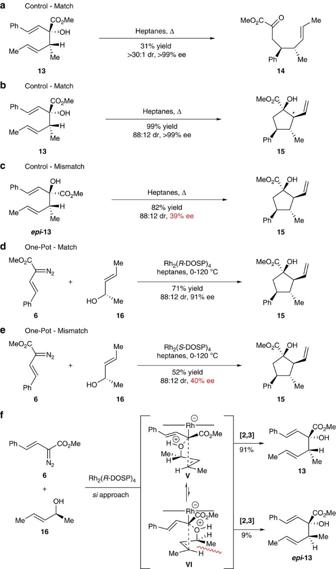Figure 5: Control studies relevant to the synthesis of cyclopentane15. (a) Chirality transfer control for the oxy-Cope rearrangement. Matched (b) and mismatched (c) tandem oxy-Cope rearrangement hetero-ene reactions of stereoisomerically pure 3-hydroxy-1,3-hexadienes (13andepi-13, respectively). Matched (d) and mismatched (e) one-pot cyclopentane (15) syntheses. (f) Justification for high, but imperfect, diastereocontrol during the rhodium-catalysed ylide formation/[2,3]-sigmatropic rearrangement. Figure 5: Control studies relevant to the synthesis of cyclopentane 15 . ( a ) Chirality transfer control for the oxy-Cope rearrangement. Matched ( b ) and mismatched ( c ) tandem oxy-Cope rearrangement hetero-ene reactions of stereoisomerically pure 3-hydroxy-1,3-hexadienes ( 13 and epi -13 , respectively). Matched ( d ) and mismatched ( e ) one-pot cyclopentane ( 15 ) syntheses. ( f ) Justification for high, but imperfect, diastereocontrol during the rhodium-catalysed ylide formation/[2,3]-sigmatropic rearrangement. Full size image In order for the Cope rearrangement to proceed with high enantiocontrol, the two chiral centres of the hexadiene must cooperatively reinforce a single chair-like transition state, as illustrated in Fig. 5a and b . In the negative control reaction with the epimeric material epi -13 , the two chiral centres are orientated competitively , such that only the carbomethoxy or the methyl group can occupy an equatorial position in the two available chair-like forms ( Fig. 5c ). The reaction with epi -13 demonstrated the detrimental effect on enantiocontrol, as the cyclopentane 15 was obtained with considerable racemization (39% ee) because of competing chair-like transition states. The identical diastereomeric ratio of product cyclopentanes observed for the matched and mismatched reactions ( Fig. 5b,c ) was again consistent with a problematic carbonyl ene reaction. These studies revealed that a second stereocentre could be manipulated for enantiocontrol in the oxy-Cope rearrangement but generated new problems with regard to the diastereoselectivity of the ene reaction. The control studies revealed that the rearrangement of the hexadienol 13 to cyclopentanol 15 could be achieved under thermal conditions without the use of scandium triflate as a Lewis acid catalyst. Therefore, modified conditions were developed for the one-pot process. Rh 2 ( R -DOSP) 4 -catalysed reaction of vinyldiazoacetate 6 with the allyl alcohol 16 followed by heating of the crude mixture for 24 h afforded the desired product in a gratifying 71% yield ( Fig. 5d ). While the diastereomeric ratio for the one-pot process was identical to that for the control reaction shown in Fig. 5b , an unanticipated decrease in the level of enantioselectivity was observed in the matched reaction to form 15 . The level of enantioselectivity was 91% ee, which is an improvement over our previous studies [52] , but still not ideal. The one-pot mismatched reaction ( Fig. 5e ), conducted by implementing the opposite enantiomer of catalyst [Rh 2 ( S -DOSP) 4 ], resulted in an overall less efficacious synthesis of 15 , as expected. The enantioselectivity of the transformation was consistent with that observed during the tandem oxy-Cope/ene study ( Fig. 5c ). The discrepancy in enantioselectivity for the cyclopentane formation in the Cope/ene sequence ( Fig. 5b ) versus the complete one-pot sequence ( Fig. 5d ) is attributed to a slight diasteromeric ‘leakage’ occurring during the [2,3]-sigmatropic rearrangement ( Fig. 5f ). In our previous study, we rationalized the driving force for diastereoselection in the ylide formation/[2,3] rearrangement to be minimization of A 1,3 -strain in the ylide intermediate. While the strain-minimized transition state V is preferred, for the pentenol 16 , the epimeric product ( epi -13 ) is also formed ( 13 : epi -13 ratio, ~11: 1) because the strain formed between a syn -pentane methyl and hydrogen group in transition state VI is not severe. According to the control study described in Fig. 5c , the minor [2,3]-product epi -13 will contribute to formation of the enantiomer of 15 . Another challenge with the second-generation substrates was the formation of diastereomers during the ene reactions. The modest level of diastereoselectivity in this step can be rationalized by a transition state analysis. Placing the ene and enophile components of 14 in a syn orientation to allow for requisite orbital overlap renders two feasible transition states ( Fig. 6a , VII and VIII ). As with the [2,3]-sigmatropic rearrangement, minimization of A 1,3 -strain is a governing factor in the carbonyl ene reaction. Since the ene consists of a trans -1,2-disubstituted alkene, the origins of any A 1,3 -strain are from interaction between the vinylic proton and the pseudoequatorial allylic methyl group. Interestingly, a similar strain interaction occurring during the [2,3]-rearrangement ene reactions produces similar levels of diastereoselectivity. Thus, while diastereomer 15 arising from cyclization via VII is preferred, some of the product epi -15 originating from the slightly more strained transition state VIII are also formed. 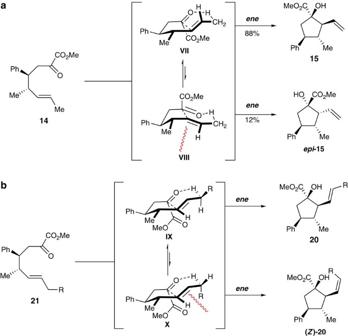Figure 6: Rationale for diastereoselectivities in the hetero-ene reaction. (a) Envelope-like transition statesVIIandVIIIfor the formation of15andepi-15, respectively. (b) Rotational isomers of an ene transition stateIXandXfor the formation of20and (Z)-20, respectively. Figure 6: Rationale for diastereoselectivities in the hetero-ene reaction. ( a ) Envelope-like transition states VII and VIII for the formation of 15 and epi- 15 , respectively. ( b ) Rotational isomers of an ene transition state IX and X for the formation of 20 and ( Z ) -20 , respectively. Full size image These studies verified both the feasibility of generating cyclopentanes in high levels of enantioselectivity via a one-pot process and the necessity of matching catalyst and alcohol chirality. We decided to explore whether the trend we observed with the allyl alcohol 16 would be extended to other secondary allyl alcohols. The diazoacetate 6 was chosen as the standard carbene precursor as it has been studied extensively in tandem ylide formation/[2,3]-sigmatropic rearrangement chemistry [52] , [55] , [68] , [69] . We found that incorporating superstoichiometric quantities of calcium chloride enabled a 10-fold reduction in the loading of dirhodium tetracarboxylate catalyst without any loss in asymmetric induction and, therefore, it was incorporated as part of the standard reaction conditions. We believe CaCl 2 helps to minimize competitive coordination of the alcohol to the vacant axial site of the dirhodium tetracarboxylate catalyst, a process that impedes denitrogenative decomposition of the diazoacetate (see Supplementary Table 1 ). The first series of alcohols ( 17a – d ) examined, similar to those in our previous cyclopentane synthesis [52] , varied in carbinol substitution ( Table 1 ). We envisioned that an increase in steric bulk at the carbinol (compared with 16 ) could enhance the diastereoselectivity of the [2,3]-sigmatropic rearrangement and, therefore, the overall enantioselectivity of the cyclopentane synthesis. Increasing the length of the alkyl chain (entries 1–2, 17a – b ) had no effect on the stereocontrol of the reaction. Introduction of more encumbered secondary carbon or benzylether substituents (entries 3–4, 17c – d , respectively) adjacent to the carbinol provided comparable yields and levels of enantioselectivity with a slight improvement in the levels of diastereoselectivity. Table 1 *Variations in carbinol substitution. Full size table We then explored the effect of increasing the bulk of the alcohol C(3) substitituent, which participates in A 1,3 interactions during the [2,3]-sigmatropic rearrangement. A modest improvement in enantioselectivity was observed when a C(3)-Me substituent ( Fig. 5d , 16 ) was replaced by an iso propyl moiety ( Table 2 , entry 1, 19a , R 1 = R 2 =Me). The diastereoselectivity, however, was similar to that observed for the previous class of allyl alcohols. For alcohols where R 1 and R 2 were not equivalent, an added element of complexity in the form of olefin geometry was introduced (entries 2–4, 19b – d ). The yields and levels of stereoselectivity were fairly consistent throughout the group; however, ( E )-selective alkene formation was correlated with the size of R 1 . Specifically, linear alkyl chains ( 19b – c ) provided comparable ratios of E - and Z diastereomers (entries 2–3, ca . 3:1, E : Z ), but a benzyl substituent afforded cyclopentane ( E )- 20d in greater than 7:1 E / Z mixture. Table 2 *Variations in allylic substitution. Full size table The preference for the formation of the E -isomers of 20 is consistent with the transition state model presented for the ene reaction as illustrated in Fig. 6b . Minimization of A 1,3 interactions dictates the major reaction pathway. By rotating the methylene carbon of the ene fragment ( Fig. 6b , IX versus X ), the allylic R-group would be positioned either trans or cis to the vinylic proton. The former, less strained intermediate would give rise to the ( E )-cyclopentane 20 , and the latter to the less preferred ( Z ) -20 . On the basis of the experimental observations and the transition state analysis, it became apparent that a highly stereoselective entry to the cyclopentanes would require effective control of chair transition states in the oxy-Cope rearrangement and maximization of the A 1,3 -strain control in the [2,3]-sigmatropic rearrangement and the ene reaction. Therefore, we examined a series of alcohols 23 bearing geminal disubstitution at the C(3) position ( Table 3 ). One of the substituents was methyl to maximize chair selectivity in the oxy-Cope rearrangement and to minimize the formation of isomers in the ene reaction. The desired chiral alcohols ( 23 ) were readily prepared from commercially available enals or by means of carbometallation [68] , [70] of the requisite alkynes and trapping with acetaldehyde. The results of the cyclopentane formation from 23 are described in Table 3 . In each case the reaction proceeds in very high yield (85–89%) and with excellent levels of stereoselectivity. The cyclopentanes 24 were formed in >30:1 dr and in 99% ee. The reaction is likely to be applicable to a range of vinyldiazoacetates as the alkyl-substituted vinyldiazoacetate ( 22 , R =Et) was similarly effective in the net transformation. The absolute configuration of cyclopentane 24a was verified by X-ray crystallographic analysis and this assignment was applied to the other products by analogy. Moreover, the absolute configuration was consistent with the assignments in our earlier studies [58] . Table 3 *Variations in vinylic substitution. Full size table Although the cyclopentane bearing a quaternary hydroxycarbonyl stereocentre is a common structural motif among numerous polyterpenoid natural products (for example, jatrophane diterpenoids), we sought to demonstrate the ease with which the products could be converted to the corresponding cyclopentanones. To this end, reduction of the cyclopentane carboxylate to the 1,2-diol was affected by lithium borohydride. Quenching with pH 7.0 buffer followed by direct treatment of the crude reaction mixture with excess sodium periodate furnished the cyclopentanone 25 in good yield with no observable epimerization of the α -stereocentre ( Table 3 ). A detailed summary and analysis of the processes involved for stereoselective synthesis of ( R,R,R,S )-28 from alcohols such as 23 is presented in Fig. 7 . The four discrete steps involved are the following: oxonium ylide formation ( Step 1 ), [2,3]-sigmatropic rearrangement ( Step 2 ), oxy-Cope rearrangement ( Step 3 ) and carbonyl ene reaction ( Step 4 ). 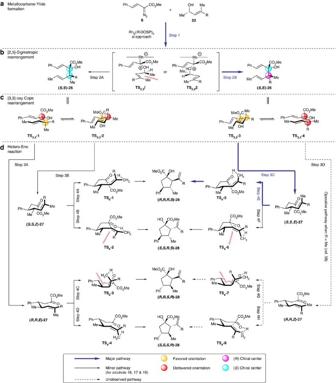Figure 7: Plausible reaction pathways in the cyclopentane synthesis.  Figure 7: Plausible reaction pathways in the cyclopentane synthesis. Full size image The reaction sequence commences with nucleophilic addition of 23 to the rhodium-bound carbene intermediate derived from diazoacetate 6 . A high degree of enantiocontrol is exerted by the rhodium catalyst, dictating si approach to the metallocarbene [58] , [68] , [69] . Thererfore, the analysis shown in Fig. 7 is limited to compounds generated from the si face attack. Due to the severe A 1,3 -strain that develops between the allylic methyl substituents in TS 2,3 1 , the reaction proceeds selectively through TS 2,3 2 , affording the hexadiene diastereomer ( S,R )-26 . Rendering the reaction intermediate into a chair-like transition state produces TS 3,3 3 , where the bulkiest substituents (CO 2 Me and R) are occupying equatorial positions. Proceeding through an oxy-Cope rearrangement with tandem enol—keto tautomerization provides the α-ketoester ( S,S,E )-27 . As with the [2,3]-sigmatropic rearrangement, the driving force for diastereoselectivity in the carbonyl ene reaction is minimization of A 1,3 interactions. Thus, the transition state where the allylic methyl groups are oriented on opposite faces of the ensuing cyclopentane ( TS e -5 ) is the dominant pathway. The result is the formation of the observed stereoisomer of the cyclopentane ( R,R,R,S )-28 . In our previous study where the [2,3]-sigmatropic rearrangement products lacked a second stereocentre ( 26 , R =Me), the 1,5-hexadiene is forged with excellent enantiocontrol. Nonetheless, during the oxy-Cope rearrangement TS 3,3 -4 becomes a viable, albeit minor, reaction pathway to give rise to ( R,R )-27 (R=Me). Since the allylic (ene) portion of the molecule is trisubstitued, it is still able to exploit a high degree of A 1,3 -strain, resulting in dramatic preference for carbonyl ene reaction through TS e 8 rather than TS e 7 . As a result, the enantiomeric cyclopentane ( S,S,S,R )-28 is formed competitively, resulting in moderate enantiomeric excess for the overall synthesis. When the allylic alcohol was not 3,3-disubstituted (for example, 16 , 17 , and 19 ), TS 2,3 1 becomes viable in the 2,3-sigmatropic rearrangement leading to the formation of some of the enantiomeric products ( S,S,S,R )-28 . In addition, TS e 2 becomes viable in the ene reaction leading to the formation of some of the diastereomeric products ( S,S,R,S )-28. Thus, a domino reaction of rhodium vinylcarbenes and enantiopure allyl alcohols provides a convergent strategy for the synthesis of cyclopentane carboxylates. Employing just 0.1 mol % of chiral catalyst, three new bonds are formed while installing four contiguous stereocentres in high yield with excellent diastereo- and enantioselectivity. A range of functional groups can be introduced at three of the stereogenic centres by variations in the allyl alcohol and vinyldiazoacetate. The fourth hydroxyester stereocentre is readily manipulated to generate complex cyclopentanones via a one-pot reduction/oxidation procedure. Each discrete step in the reaction sequence involves distinct chirality-transfer events, which can be manipulated by appropriate substitution of the alcohol and ensuing intermediates. A detailed understanding of the stereochemical processes involved in the cascade has been developed, allowing for exceptional control over each stereochemical transfer. The low catalyst loadings, readily available starting materials and in-depth understanding of the mechanistic details make this an attractive method for accessing substituted cyclopentanes. General considerations All reactions were conducted in oven-dried glassware under an inert atmosphere of dry argon. All chemicals were purchased from either Sigma-Aldrich, TCI America, Acros or Alfa-Aesar and were used as received. Pentane, hexanes, tetrahydrofuran and diethyl ether were obtained from a Grubbs-type solvent purification system. Heptanes were purchased from Macron Fine Chemicals and were used as received. Calcium chloride was dried at 200 °C under vacuum for 12 h and stored in a dessicator. 1 H NMR spectra were recorded at either 400 MHz on an INOVA-400 spectrometer or at 600 MHz on an INOVA-600 spectrometer. 13 C NMR spectra were recorded at 100 MHz on an INOVA-400 spectrometer. NMR spectra were recorded in deuterated chloroform (CDCl3) solutions, with residual chloroform ( δ 7.27 p.p.m. for 1 H NMR and δ 77.23 p.p.m. for 13 C NMR) or tetramethylsilane ( δ 0.00 p.p.m. for 1 H NMR) taken as the internal standard, and were reported in p.p.m. Abbreviations for signal coupling are as follows: s, singlet; d, doublet; t, triplet; q, quartet; m, multiplet. Coupling constants were taken from the spectra directly and are uncorrected. IR spectra were collected on a Nicolet iS10 FT-IR spectrometer as neat films. Mass spectrum determinations were carried out on a Thermo Finnigan LTQ-FTMS spectrometer with electrospray or atmospheric pressure chemical ionization. Optical rotations were measured on JASCO P-2000 polarimeter. Gas chromatography (GC) analysis was performed on an Agilent 7890A; column conditions: 30 °C for 1 min, then increasing to 180 °C at a rate of 5 °C min −1 , then 180 °C for 5 min. Analytical thin layer chromatography was performed on silica gel plates using UV. For details of chromatography and previously reported syntheses of substrates 2 , Rh 2 ( S -DOSP) 4 and Rh 2 ( R -DOSP) 4 , 16 , 17b–d , 19a and c , 23b , 17a , 19b , 19d , and 23a , see Supplementary Methods. For 1 H and 13 C NMR data see Supplementary Figs 3–34 . For HPLC traces, see Supplementary Figs 35–47 . For an ORTEP diagram of compound 24a, see Supplementary Fig. 48 . General procedure A 35-ml pressure tube fitted with a rubber septum was evacuated and backfilled with dry Ar (3 × ). The reaction vessel was charged with Rh 2 ( R -DOSP) 4 (0.9 mg, 0.005 mmol, 0.1 mol %) and anhydrous CaCl 2 (111 mg, 1.0 mmol, 2.0 equiv) before adding a heptane solution (1.0 ml) of 16 (43 mg, 0.50 mmol, 1.0 equiv). The suspension was cooled to 0 °C in an ice bath. A heptane solution (5 ml) of 6 (121 mg, 0.60 mmol, 1.2 equiv) was added dropwise over 0.5 h accompanied by vigorous stirring. The reaction was further stirred at 0 °C for 2 h, before removing the ice bath and allowing to warm to ambient temperature. The rubber septum was removed and the vessel was sealed with a Teflon screwcap. The sealed tube was immersed in an oil bath preheated to 125 °C. After 48 h, the reaction was cooled to ambient temperature and the suspension was filtered through a fritted glass funnel, washing the filter cake with pentane (3 × 10 ml), and the filtrate was concentrated in vacuo . Column chromatography (SiO 2 , pentane/diethyl ether, 10:1) afforded a single diastereomer of the pure product 15 (92 mg, 71% yield). For additional procedures see Supplementary Methods . Accession codes : The X-ray crystallographic coordinates for structure 24a have been deposited at the Cambridge Crystallographic Data Centre (CCDC), under deposition number CCDC 955223. These data can be obtained free of charge from The Cambridge Crystallographic Data Centre via www.ccdc.cam.ac.uk/data_request/cif. How to cite this article: Parr, B. T. and Davies, H. M. L. Highly stereoselective synthesis of cyclopentanes bearing four stereocentres by a rhodium carbene-initiated domino sequence. Nat. Commun. 5:4455 doi: 10.1038/ncomms5455 (2014).